Trim71 cooperates with microRNAs to repress Cdkn1a expression and promote embryonic stem cell proliferation Pluripotent embryonic stem cells have a shortened cell cycle that enables their rapid proliferation. The embryonic stem cell-specific miR-290 and miR-302 microRNA families promote proliferation whereas let-7 microRNAs inhibit self-renewal, and promote cell differentiation. Lin28 suppresses let-7 expression in embryonic stem cells. Here to gain further insight into mechanisms controlling embryonic stem cell self-renewal, we explore the molecular and cellular role of the let-7 target Trim71 (mLin41). We show that Trim71 associates with Argonaute2 and microRNAs, and represses expression of Cdkn1a, a cyclin-dependent kinase inhibitor that negatively regulates the G1–S transition. We identify protein domains required for Trim71 association with Argonaute2, localization to P-bodies, and for repression of reporter messenger RNAs. Trim71 knockdown prolongs the G1 phase of the cell cycle and slows embryonic stem cell proliferation, a phenotype that was rescued by depletion of Cdkn1a. Thus, we demonstrate that Trim71 is a factor that facilitates the G1–S transition to promote rapid embryonic stem cell self-renewal. Embryonic stem cells (ESCs) have the capacity to self-renew indefinitely and, being pluripotent, can differentiate to specialized cell types. Rapid ESC self-renewal is achieved by an expedited cell cycle with a shortened G1 phase. microRNAs (miRNAs) have recently emerged as important regulators of cell fate decisions and have a key role in mediating this unique cell-cycle structure in ESCs. These ~22 nucleotide (nt) regulatory RNAs function to guide the miRNA-induced silencing complex (miRISC) to complementary sites in target messenger RNAs for posttranscriptional gene repression by translational repression and/or mRNA degradation [1] . Members of the Argonaute (Ago) and the GW182 families of proteins have been identified as essential components of miRISC, localize to cytoplasmic P-bodies, and act as key effectors in miRNA function [2] , [3] , [4] . Mouse and human ESCs express a limited repertoire of miRNAs whose levels decrease as the cells differentiate [5] . Members of mouse ESC-specific miR-290 family (miR-290, miR-291a, miR-291b, miR-292, miR-293, miR-294, miR-295) and miR-302 family (miR-302a, miR-302b, miR-302c, miR-302d, miR-367) share similar seed sequences (and likely function redundantly to repress a common set of targets), and can rescue the proliferation defects of miRNA-deficient ESCs by suppressing several key regulators of the G1–S phase transition [6] , [7] . Introduction of let-7 miRNAs into miRNA-deficient ESCs can rescue their compromised differentiation presumably by directly downregulating key pluripotency factors [7] , [8] , [9] . The let-7 family comprises 12 members with a conserved seed sequence. Let-7 is highly expressed in differentiated cells and tissues and its expression is tightly regulated during ESC differentiation by the RNA-binding protein Lin28 and its associated 3′ terminal uridylyl transferase Zcchc11 (TUT4) that prevents let-7 biogenesis in undifferentiated ESCs [10] , [11] , [12] . Altogether, the current model suggests that the different families of miRNAs control the self-renewal and differentiation of ESCs. The Lin28-let-7 regulatory feedback loop is conserved in Caenorhabditis elegans , and lin-41 is a heterochronic gene whose expression is directly regulated by let-7 in C. elegans. lin-41 encodes a member of the Trim-NHL family [13] , [14] . Trim-NHL proteins contain multiple tandem repeats of a carboxy-terminal NHL domain, a coiled-coil region, one or more B-boxes, and sometimes an amino-terminal RING finger. The Trim-NHL (and NHL-only) family represents an evolutionarily conserved set of genes that are critical for a variety of cell fate transitions [15] , [16] . lin-41 loss-of-function mutations induce precocious expression of adult cell fates at larval stages [17] . Ectopic lin-41 activity causes the opposite phenotype, reiteration of larval cell fates. lin-41 expression is post-transcriptionally downregulated at late larval stages by let-7 and lin-4 miRNAs [14] . Although the molecular function of LIN-41 is largely unknown, LIN-41 was identified as a DCR-1-interacting protein [18] . Trim71, the mammalian homologue of LIN-41, is highly expressed during early mouse embryogenesis and is downregulated at mid-embryogenesis when let-7 and mir-125 (orthologue of lin-4 ) levels are induced [19] . Genetic perturbations of Trim71 in mice [20] and zebrafish cause embryonic lethality, indicating an essential role of Trim71 in normal development [19] , [21] . Finally, a report identified Trim71 as an E3 ubiquitin ligase for Ago2 (ref. 22 ). In C. elegans , certain other Trim-NHL genes, including nhl-2 , are essential for normal developmental timing [23] . In Drosophila , the tumour suppressors, Brat and Mei-P26, inhibit the self-renewal capability of stem cells from neuronal and ovarian lineages, respectively [24] , [25] , [26] . Mutations of the tumour suppressor dappled cause a melanotic tumour phenotype, and hence Dappled is also likely involved in cell proliferation control [27] . In mice, Trim32 prevents self-renewal and promotes differentiation in neural progenitors [28] . Importantly, several of the aforementioned Trim-NHL proteins physically interact with Ago proteins and have been functionally implicated in miRNA-mediated gene regulation [23] , [25] , [28] . For example, Mei-P26 reportedly inhibits miRNA expression [25] . However, other Trim-NHL proteins, including NHL-2 and Trim32, enhance the function of certain miRNAs without affecting miRNA levels [23] , [28] . For instance, NHL-2 enhances the post-transcriptional repression of let-7 targets [23] . Therefore, Trim-NHL proteins seem to control miRNA activity by more than one mechanism. Here we investigated the molecular and cellular function of Trim71 (mLin41) in mouse ESCs and identify Trim71 as a miRISC-interacting protein. We confirm that Trim71 interacts with Ago2 and extend these studies by identifying the domains of Trim71 protein required for this interaction and for Trim71 localization to P-bodies. We find that Trim71 functionally interacts with ESC-specific miRNAs to post-transcriptionally repress expression of the cell cycle regulator Cdkn1a. We furthermore demonstrate that, when directly tethered to mRNA, Trim71 can post-transcriptionally repress expression of a reporter and we dissect the protein domains mediating this repression. Knockdown of Trim71 prolongs the G1 phase of the cell cycle and slows ESC proliferation, a phenotype that is rescued by depletion of Cdkn1a. Our study identifies Trim71 as a factor that facilitates the G1–S transition to promote rapid ESC proliferation and highlights the importance of miRNA gene regulatory networks in the balance between stem cell self-renewal and differentiation. Trim71 is highly expressed in undifferentiated ESCs We examined the relative expression of Trim71 in mouse ESCs and several differentiated cell and tissue types and found that Trim71 is highly expressed in undifferentiated ESCs (J1) and embryonal carcinoma (EC) cells (P19), but not expressed in any of the differentiated cells and tissues examined ( Fig. 1a ). Similarly, Trim71 protein was readily detected in ESCs and EC cells, but not in mouse fibroblasts (NIH 3T3) ( Fig. 1b ). In embryoid body-formation assays Trim71 and the pluripotency factor Oct-4 were downregulated on cell differentiation ( Fig. 1c ) [29] . During the course of cell differentiation, let-7 g was upregulated whereas miR-295 was downregulated ( Fig. 1c ). Previously, we found that the developmentally regulated RNA-binding protein Lin28 functions in ESCs to inhibit the maturation of let-7 miRNAs [10] , [11] , [12] , [30] . As the 3′-UTR of human Trim71 contains two validated let-7 target sites [21] , we explored the relationship between Lin28 and Trim71 expression in mouse ESCs. Knockdown of Lin28 led to a dramatic increase in the levels of let-7 family members and a concomitant decrease in the levels of Trim71, an effect that was suppressed by a let-7 inhibitor ( Fig. 1d-f ). Lin28 depletion did not result in changes in Sox2, Nanog, or Oct4 expression during the time course of this experiment, indicating that the observed decrease in Trim71 expression is unlikely a result of cell differentiation ( Fig. 1d ). Conversely, depletion of Trim71 had no obvious effect on Lin28 levels or Sox2, Nanog, or Oct4 expression. A luciferase reporter containing let-7 binding sites from the Trim71 3′-UTR, but not a control reporter, was repressed in cells that express high levels of endogenous let-7 ( Fig. 1g ). Reporter activity was de-repressed on treatment with anti-let-7a but not a control miRNA inhibitor. Altogether, our results demonstrate that mouse Trim71 is a bona fide let-7 target downstream of Lin28. 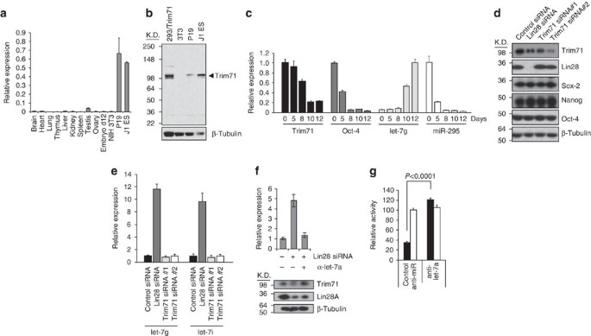Figure 1: Trim71 is highly expressed in undifferentiated cells and is a let-7 target. (a) qRT–PCR of Trim71 mRNA levels (normalized to β-actin levels). (b) Western blot of Trim71 protein (arrowhead) using a rabbit polyclonal antibody. Flag-Trim71 expressed in HEK293 cells serves as a positive control. β-tubulin was used as a loading control. (c) qRT–PCR for Oct-4 and Trim71 (normalized to β-actin) and TaqMan qRT–PCR for mature let-7 g and miR-295 (normalized to snoRNA142) during ESC differentiation to embryoid bodies. RNA was prepared from V6.5 ESCs on day 0 (undifferentiated) and on day 5, 8, 10 and 12 of differentiation. (d) Whole-cell extracts from J1 ESCs transfected with control, Lin28 or Trim71 siRNA were examined by western blot 60 h post-transfection. (e) TaqMan PCR of mature let-7 levels from samples in (d). (f) Samples from J1 ESCs transfected with Lin28 siRNA, anti-let-7a, or both were examined by TaqMan PCR for mature let-7a (top) and by western blot (bottom). (g) Luciferase reporter assays performed in HeLa cells using a firefly luciferase that contains two let-7-binding sites from the mouse Trim71 3′-UTR. All Signals were normalized to Renilla luciferase levels. Error bars represent mean+/−s.d. withn=3. TheP-value is from a two-tailedt-test. Figure 1: Trim71 is highly expressed in undifferentiated cells and is a let-7 target. ( a ) qRT–PCR of Trim71 mRNA levels (normalized to β-actin levels). ( b ) Western blot of Trim71 protein (arrowhead) using a rabbit polyclonal antibody. Flag-Trim71 expressed in HEK293 cells serves as a positive control. β-tubulin was used as a loading control. ( c ) qRT–PCR for Oct-4 and Trim71 (normalized to β-actin) and TaqMan qRT–PCR for mature let-7 g and miR-295 (normalized to snoRNA142) during ESC differentiation to embryoid bodies. RNA was prepared from V6.5 ESCs on day 0 (undifferentiated) and on day 5, 8, 10 and 12 of differentiation. ( d ) Whole-cell extracts from J1 ESCs transfected with control, Lin28 or Trim71 siRNA were examined by western blot 60 h post-transfection. ( e ) TaqMan PCR of mature let-7 levels from samples in ( d ). ( f ) Samples from J1 ESCs transfected with Lin28 siRNA, anti-let-7a, or both were examined by TaqMan PCR for mature let-7a (top) and by western blot (bottom). ( g ) Luciferase reporter assays performed in HeLa cells using a firefly luciferase that contains two let-7-binding sites from the mouse Trim71 3′-UTR. All Signals were normalized to Renilla luciferase levels. Error bars represent mean+/−s.d. with n =3. The P -value is from a two-tailed t -test. Full size image Trim71 is an Ago2-interacting protein To explore whether Trim71 can physically interact with Ago proteins in ESCs, we generated a stable mouse ESC line (KH2) for doxycycline (Dox)-inducible Flag-Trim71 expression. Large-scale Flag-immunoprecipitation (IP) followed by mass spectrometry identified Ago2 along with other members of the Ago family as Trim71-associated proteins (data not shown). Co-immunoprecipitation assays in ES, HEK293, and EC cells confirmed that Trim71 specifically associates with Ago2 ( Fig. 2a-c ). We found this interaction to be salt-sensitive and RNA dependent ( Fig. 2a ). To confirm the efficacy of RNase treatment in these experiments, we examined the expression of ESC miRNAs in control and treated extracts, and found mature miRNAs were effectively depleted by RNase treatment ( Fig. 2b ). We also performed western blot analysis on these samples and found levels of Ago2 protein to be unchanged, thereby further supporting an RNA-dependent interaction between Trim71 and Ago2 ( Fig. 2b ). To investigate the reciprocal interaction between Ago2 and Trim71, we generated another stable mouse ESC line for Dox-inducible expression of Flag-Ago2. We detected endogenous Trim71 in Flag-Ago2 but not control Flag-Lin28 affinity eluates ( Fig. 2d ). Finally, we also confirmed a physical interaction between endogenous Trim71 and Ago2 proteins in ESCs ( Fig. 2e, f ). Together, we confirm that Trim71 is an Ago2-associated factor in ESCs. 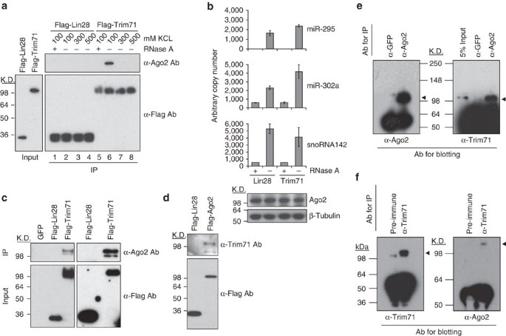Figure 2: Trim71 interacts with Argonaute2. (a) Cell extracts were prepared from KH2 ESCs expressing either Flag-Lin28 or Flag-Trim71. Flag-affinity purifications were washed with buffer containing the indicated KCl concentration. Where indicated, RNase A was added to the lysates for IP. The input and affinity eluates were analysed by western blot. (b) Analysis of miRNA and Argonaute protein in RNase-treated extracts. TaqMan qRT–PCR for the indicated miRNA (Top), Error bars represent mean+/−s.d. withn=3, and western blot for Ago2 (bottom). (c) Flag-affinity purifications on whole-cell extracts from HEK293 (left) and P19 (right) that were transfected to express Flag-Trim71 or the indicated control proteins. Western blots performed using α-Flag and α-Ago2 antibodies. (d) Flag IPs performed as in (a) (100 mM KCl washes). The eluates were analysed by western blot. (e,f) Endogenous co- immunoprecipitation from J1 whole-cell extracts performed with the indicated antibodies. The immunoprecipitated proteins are indicated by arrowheads. Figure 2: Trim71 interacts with Argonaute2. ( a ) Cell extracts were prepared from KH2 ESCs expressing either Flag-Lin28 or Flag-Trim71. Flag-affinity purifications were washed with buffer containing the indicated KCl concentration. Where indicated, RNase A was added to the lysates for IP. The input and affinity eluates were analysed by western blot. ( b ) Analysis of miRNA and Argonaute protein in RNase-treated extracts. TaqMan qRT–PCR for the indicated miRNA (Top), Error bars represent mean+/−s.d. with n =3, and western blot for Ago2 (bottom). ( c ) Flag-affinity purifications on whole-cell extracts from HEK293 (left) and P19 (right) that were transfected to express Flag-Trim71 or the indicated control proteins. Western blots performed using α-Flag and α-Ago2 antibodies. ( d ) Flag IPs performed as in ( a ) (100 mM KCl washes). The eluates were analysed by western blot. ( e , f ) Endogenous co- immunoprecipitation from J1 whole-cell extracts performed with the indicated antibodies. The immunoprecipitated proteins are indicated by arrowheads. Full size image Trim71 associates with miRNAs and catalytically active Ago2 In light of an RNA-dependent interaction between Trim71 and Ago2 proteins in ESCs, we hypothesized that Trim71 may also be associated, albeit indirectly, with ESC-specific miRNAs. To test this, we immunoprecipitated Flag-Trim71 from ultraviolet-crosslinked Dox-inducible ESCs, isolated the associated RNA, and quantified levels of miRNA by quantitative real-time PCR (qRT–PCR). We found that members of the miR-290 and miR-302 families were enriched in Flag-Trim71 IP compared with a control snoRNA142 ( Fig. 3a ). When guided by miRNAs to RNAs of complementary sequence, Ago2 can mediate the endonucleolytic cleavage of the target RNA, an activity that has been dubbed 'slicer' activity. We incubated Flag-Trim71, Flag-Ago2, or control Flag-Lin28 purified from ESCs with a 5′-end-labelled target RNA that is fully complementary to a ES cell-specific miRNA (miR-295 or miR-302a). As expected, Flag-Ago2 eluate displayed strong slicing activity on both target RNAs. Interestingly, Flag-Trim71, but not Flag-Lin28, affinity-purified complex also exhibited cleavage activity on the same target RNAs ( Fig. 3b ). These experiments indicate that Trim71 associates with ribonucleoprotein complexes containing catalytically active Ago2 and functional miR-295 and miR-302 in ESCs. We postulated that the RNA-dependent interaction between Trim71 and Ago2 might be mediated by miRNA. To test this we investigated whether Trim71 can associate with a miRNA binding-deficient Ago2 protein. The ability of Ago2 to interact with miRNAs is substantially reduced by mutations in its PAZ domain [4] . We co-expressed Flag-Trim71, together with either wild-type or PAZ mutant Ago2, in ESCs and examined the association of these proteins by co-IP. Interestingly, although wild-type Ago2 was readily co-precipitated with Trim71, the Ago2-PAZ10 mutant was not detectable in the purified complex ( Fig. 3c ). Therefore, the interaction between Trim71 and Ago2 is mediated by miRNAs, supporting the notion that Trim71 may function together with miRISC. 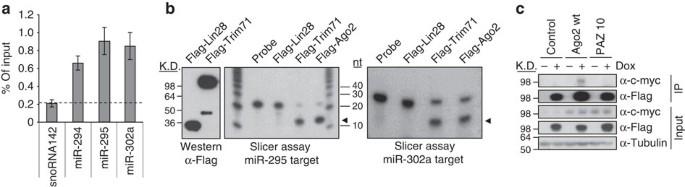Figure 3: Trim71 ribonucleoprotein complex contains miRNAs. (a) Ultraviolet crosslinking IP (CLIP) on Dox-inducible Flag-Trim71 ESCs. RNA analysis for the indicated miRNAs or control RNA performed using TaqMan qRT–PCR and the pull-down efficiency of each RNA is represented as % of input. Error bars represent mean +/−s.d. withn=3. (b) Slicer assays performed on Flag-affinity eluates (100 mM KCl washes) to monitor Ago2-mediated RNA cleavage activity. Left: western blot of the Flag-Lin28 and Flag-Trim71 IP eluates used in slicer assays. Right: reaction products resolved by 15% denaturing PAGE. Arrowhead indicates the specific 5′ cleavage product of the target RNA. (c) Flag-IP Flag-Trim71 expressing ESCs transfected with wild-type or PAZ10 Myc-Ago2 construct. Affinity eluates were probed with α-Flag and α-Myc antibodies. Figure 3: Trim71 ribonucleoprotein complex contains miRNAs. ( a ) Ultraviolet crosslinking IP (CLIP) on Dox-inducible Flag-Trim71 ESCs. RNA analysis for the indicated miRNAs or control RNA performed using TaqMan qRT–PCR and the pull-down efficiency of each RNA is represented as % of input. Error bars represent mean +/−s.d. with n =3. ( b ) Slicer assays performed on Flag-affinity eluates (100 mM KCl washes) to monitor Ago2-mediated RNA cleavage activity. Left: western blot of the Flag-Lin28 and Flag-Trim71 IP eluates used in slicer assays. Right: reaction products resolved by 15% denaturing PAGE. Arrowhead indicates the specific 5′ cleavage product of the target RNA. ( c ) Flag-IP Flag-Trim71 expressing ESCs transfected with wild-type or PAZ10 Myc-Ago2 construct. Affinity eluates were probed with α-Flag and α-Myc antibodies. Full size image The NHL domain of Trim71 mediates the interaction with Ago2 Drosophila Mei-P26, Brat, and Dappled have been shown to interact with Ago1 via their NHL domain [25] . Similarly, the NHL domain of mouse Trim32 is required for enhancement of miRNA activity [28] . In contrast, Rybak et al . reported that the coiled-coil motif of Trim71 is crucial for the interaction with Ago2 (ref. 22 ). We generated a series of N- and C-terminal deletions of Trim71 and assessed their ability to co-precipitate endogenous Ago2 ( Fig. 4 ). We found that whereas all the N-terminal truncations interact with Ago2, the C-terminal deletions are impaired in their ability to associate with Ago2. Moreover, we found that the C-terminal NHL domain alone (ΔN570) is sufficient for this association, suggesting that the NHL domain of Trim71 mediates the interaction with Ago2 ( Fig. 4 ). 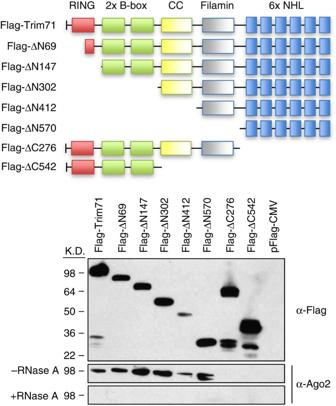Figure 4: Trim71 domains required for interaction with Ago2. Top: schematic representation of Trim71 deletion constructs. Bottom: the constructs were assessed for their ability to co-precipitate endogenous Ago2 in HeLa cells. Flag-IPs were performed in the presence or absence of RNase A. Figure 4: Trim71 domains required for interaction with Ago2. Top: schematic representation of Trim71 deletion constructs. Bottom: the constructs were assessed for their ability to co-precipitate endogenous Ago2 in HeLa cells. Flag-IPs were performed in the presence or absence of RNase A. Full size image Trim71 localizes to Processing-bodies Ago proteins localize to discrete cytoplasmic speckles designated Processing-bodies (P-bodies), which can serve as sites of translational repression, decapping- and nonsense-mediated mRNA decay, and importantly, miRNA-mediated repression [4] . By immunocytochemistry, we observed that Trim71 localizes to P-bodies in ESCs, as demonstrated by its co-localization with the mRNA-decapping enzyme DCP1a, a known P-body component ( Fig. 5a ). Similarly, we found that a mCherry::Trim71 fusion protein localizes to P-bodies in HeLa cells ( Fig. 5b ). Our observations are in accordance with the work by Rybak et al ., where Trim71 was also found localized to P-bodies [22] . To investigate the contribution of different domains of Trim71 to its subcellular localization, we examined the localization of a panel of Trim71 deletions fused to mCherry ( Fig. 5c ). We found that deletion of the RING finger (ΔN69 and ΔN147) does not affect the co-localization of Trim71 with DCP1a. In contrast, deletion of the NHL domain (ΔC276) impairs P-body localization. However, the NHL domain is not sufficient to direct P-body localization, since the ΔN570 construct fails to localize at P-bodies. We suggest that additional domains are required to direct Trim71 to P-bodies. For instance, our data indicate that deletion of the two B-boxes compromised P-body localization because only a small fraction of cells transfected with the ΔN302 or ΔN412 constructs showed P-body localization ( Fig. 5c ) whereas all the transfected cells (including those with speckles shown) display a broader cytoplasmic distribution similar to the C-terminal deletion constructs (ΔC276 and ΔC542). In agreement with our observation, Rybak et al . reported that an N-terminal truncation, deleting the RING finger and B-boxes (ΔN1-342), displays a broad cytoplasmic localization as opposed to P-body localization [22] . Altogether, our data suggest that Trim71 localizes to P-bodies in mouse ESCs, and multiple protein domains may be required for its proper subcellular localization. 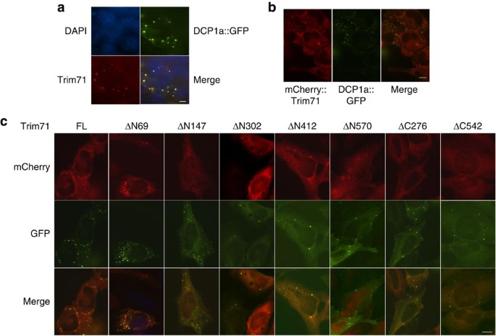Figure 5: Trim71 domains required for P-body localization. (a) KH2 ESCs transfected with a DCP1a::GFP construct are fixed and probed with α-Trim71 antibody. Nuclei are stained with DAPI. (b) HeLa cells are co-transfected with DCP1a::GFP and mCherry::Trim71 fusions. (c) Individual mCherry::Trim71 constructs were co-transfected with DCP1a::GFP into HeLa cells and visualized by fluorescence microscopy. Scale bar, 5 μm. Figure 5: Trim71 domains required for P-body localization. ( a ) KH2 ESCs transfected with a DCP1a::GFP construct are fixed and probed with α-Trim71 antibody. Nuclei are stained with DAPI. ( b ) HeLa cells are co-transfected with DCP1a::GFP and mCherry::Trim71 fusions. ( c ) Individual mCherry::Trim71 constructs were co-transfected with DCP1a::GFP into HeLa cells and visualized by fluorescence microscopy. Scale bar, 5 μm. Full size image Trim71 functions with miRNAs to repress Cdkn1a expression Our observations indicate that Trim71 interacts with catalytically active miRISC and ESC-specific miRNAs. The miRNAs from the miR-290 and miR-302 families share a very similar seed sequences and have been demonstrated to target the cell cycle regulatory gene Cdkn1a/p21 (ref. 7 ). We therefore explored Trim71 function in the context of miRNA-mediated Cdkn1a regulation in ESC. Interestingly, we found Cdkn1a protein levels increase in ESCs when Trim71 is depleted ( Fig. 6a ), a result not caused by possible cell differentiation on Trim71 knockdown as Sox2, Nanog, and Oct4 protein levels remain constant ( Fig. 1d ). Trim71 has been recently implicated in the regulation of Ago2 turnover as an E3 ubiquitin ligase [22] . However, in several independent experiments, we did not observe changes in Ago2 levels on Trim71 knockdown ( Fig. 6a , data not shown). In addition, we found no significant change in mature miR-295 and miR-302a levels ( Fig. 6b ), hence eliminating the possibility that reduced ESC-specific miRNAs and/or Ago2 levels on Trim71 depletion might account for the Cdkn1a upregulation. 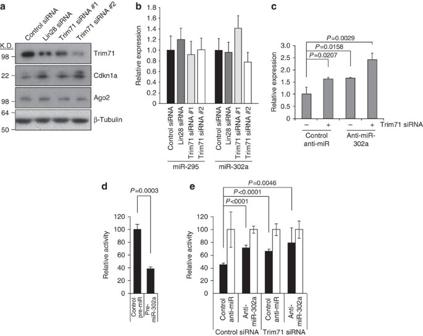Figure 6: Trim71 cooperates with miR-302 to inhibit Cdkn1a expression. (a) Trim71 depletion leads to upregulation of Cdkn1a. The same cell extracts fromFig. 1(d)were blotted with α-Cdkn1a antibody. (b) TaqMan PCR for mature miR-295 and miR-302a levels (normalized to snoRNA142). Error bars represent mean+/−s.d. withn=3. (c) J1 ESCs transfected with Trim71 siRNA or control siRNA, together with anti-miR-302a or control inhibitor, as indicated. 60 h post-transfection total RNA was analysed by qRT–PCR for Cdkn1a mRNA levels (normalized to β-actin). Error bars represent mean +/−s.d. withn=3. (d) Reporter assays were performed using a firefly luciferase that contains a miR-302 binding site from the mouse Cdkn1a 3′-UTR. A control pre-miRNA or pre-miR-302a was transfected into HeLa cells that do not express ESC-specific miRNAs. Signals were normalized to Renilla luciferase levels. Normalized signals for the pre-miR control were set to 100. (e) Reporter assays were performed 60 h post-transfection using the same luciferase constructs as in (d) as well as with a mutant reporter (white bars) in which nucleotides corresponding to the miR-302 seed sequence were mutated. Normalized signals for the mutant construct were set to 100 in each condition. Error bars represent mean +/−s.d. withn=3. TheP-values are from two-tailedt-test. Figure 6: Trim71 cooperates with miR-302 to inhibit Cdkn1a expression. ( a ) Trim71 depletion leads to upregulation of Cdkn1a. The same cell extracts from Fig. 1(d) were blotted with α-Cdkn1a antibody. ( b ) TaqMan PCR for mature miR-295 and miR-302a levels (normalized to snoRNA142). Error bars represent mean+/−s.d. with n =3. ( c ) J1 ESCs transfected with Trim71 siRNA or control siRNA, together with anti-miR-302a or control inhibitor, as indicated. 60 h post-transfection total RNA was analysed by qRT–PCR for Cdkn1a mRNA levels (normalized to β-actin). Error bars represent mean +/−s.d. with n =3. ( d ) Reporter assays were performed using a firefly luciferase that contains a miR-302 binding site from the mouse Cdkn1a 3′-UTR. A control pre-miRNA or pre-miR-302a was transfected into HeLa cells that do not express ESC-specific miRNAs. Signals were normalized to Renilla luciferase levels. Normalized signals for the pre-miR control were set to 100. ( e ) Reporter assays were performed 60 h post-transfection using the same luciferase constructs as in ( d ) as well as with a mutant reporter (white bars) in which nucleotides corresponding to the miR-302 seed sequence were mutated. Normalized signals for the mutant construct were set to 100 in each condition. Error bars represent mean +/−s.d. with n =3. The P -values are from two-tailed t -test. Full size image Our observation that Trim71 negatively regulates Cdkn1a expression supports the notion that Trim71 may cooperate with miRNAs for the post-transcriptional repression of Cdkn1a. We therefore simultaneously depleted Trim71, using short interfering RNA (siRNA), and abrogated endogenous miR-302 function, using modified antisense oligoucleotides (anti-miR-302) in ESCs. We found inhibition of miR-302 led to increased Cdkn1a expression, consistent with Cdkn1a being a direct miR-302 target ( Fig. 6c ). Similarly, knockdown of Trim71 also upregulated Cdkn1a levels. Simultaneous depletion of both miR-302 and Trim71 resulted in a further increase in Cdkn1a levels. To investigate whether Trim71-mediated Cdkn1a repression requires a functional miRNA-binding site in the Cdkn1a 3′-UTR, we cloned a 59-nucleotide fragment of the Cdkn1a 3′-UTR spanning the validated miR-302 binding site into the 3′-UTR of a firefly luciferase reporter gene. We first validated that this reporter is responsive to miR-302a levels ( Fig. 6d ). We then co-transfected the reporter together with a miR-302 inhibitor, Trim71 siRNA, or both, into ESCs ( Fig. 6e ). We found that the reporter was de-repressed by inhibition of endogenous miR-302. Knockdown of Trim71 similarly led to increased reporter gene expression. Simultaneous reduction of both miR-302 and Trim71 levels led to a further increase in the Cdkn1a reporter activity compared with a control reporter in which only the miR-302 seed sequence binding site was mutated ( Fig. 6e ). These results provide evidence that the direct repression of Cdkn1a expression by Trim71 requires an intact miR-302-binding site. Our data strongly suggest that Trim71 cooperates with ESC-specific miRNAs including miR-302 to directly repress Cdkn1a. Trim71 inhibits gene expression post-transcriptionally We next explored whether Trim71 can mediate post-transcriptional gene repression. We exploited a tethering methodology in which a protein of interest is brought to the 3′-UTR of a luciferase reporter through a heterologous RNA–protein interaction. Specifically, a MS2-fusion protein is co-expressed with a luciferase reporter construct containing high-affinity MS2-binding sites in its 3′-UTR. GW182 proteins function with Ago proteins to induce miRNA-mediated repression. Vertebrates possess three GW182 paralogues: TNRC6A, B and C. The C-terminal domain of these proteins is sufficient to mediate post-transcriptional repression in tethering assays [31] , [32] . In contrast, another P-body component Rck is reported not to mediate repression in tethering assays [32] . We constructed a MS2–Trim71 fusion as well as MS2-TNRC6B C-terminus and MS2-Rck (as positive and negative controls, respectively) [32] . We found that, while MS2-Rck exhibits no inhibitory effect, MS2-TNRC6B C-terminus inhibits reporter expression in wild-type ESCs. As any requirement for RNA interaction is bypassed in the tethering methodology, MS2-TNRC6B C-terminus also exhibits reporter repression in miRNA-deficient ESCs ( Fig. 7a ). Interestingly, MS2–Trim71 also displays significant repression of reporter expression in both cell types. Neither TNRC6B C-terminus nor Trim71 represses the reporter activity when not tethered to its transcript, arguing that their inhibitory effects are specific to the associated RNA ( Fig. 7b ). To gain further insight into the Trim71 domains required for this post-transcriptional gene silencing (PTGS), we generated a panel of additional constructs in which various Trim71 deletions (as in Fig. 4 ) were fused to MS2 and tested these deletion mutants in tethering assays. This analysis revealed that though the N-terminal RING finger and B-Boxes, as well as the C-terminal NHL domain are dispensable for PTGS, constructs lacking the coiled-coil region did not repress the reporter in these tethering assays ( Fig. 7c ). These results identify the coiled-coil as the domain of Trim71 necessary for PTGS. Altogether, our results dissect the distinct Trim71 domain requirements for Ago2-interaction, P-body localization, and for PTGS ( Fig. 7d ). 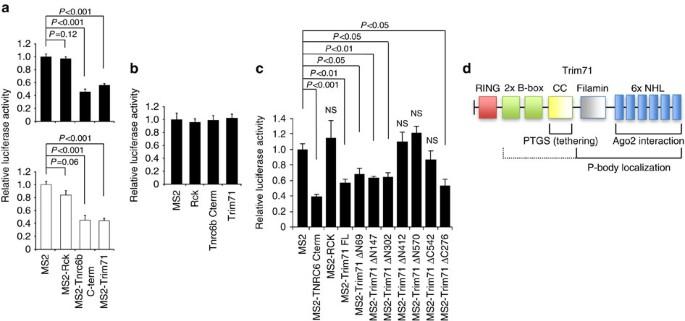Figure 7: Post-transcriptional gene repression by Trim71. (a) Tethering assays. Wild-type (upper panel) and DGCR8 KO (lower panel) ESCs were transfected with a Renilla luciferase, a firefly luciferase with or without MS2-binding sites in the 3′-UTR, and a plasmid expressing either MS2 protein or MS2-fusion, as indicated. Firefly/Renilla ratios were calculated. Relative luciferase activity represents the ratio of the reporter containing MS2-binding sites to the reporter lacking a site. Normalized signals for the MS2 control were set to 1 (b) Tethering assays in wild-type V6.5 ESCs were performed as in (a) except Rck, TNRC6B, or Trim71 not fused to MS2 (and hence not tethered to the firefly luciferase mRNA 3′-UTR). (c) Tethering assays in Hela cells performed as in (a) with the indicated Trim71 deletion MS2 fusion proteins. Normalized signals for the MS2 control were set to 1. Error bars represent mean +/−s.d. withn=3. TheP-values are from two-tailedt-test result. NS = not significant. (d) Schematic representation of functional domains of Trim71. Figure 7: Post-transcriptional gene repression by Trim71. ( a ) Tethering assays. Wild-type (upper panel) and DGCR8 KO (lower panel) ESCs were transfected with a Renilla luciferase, a firefly luciferase with or without MS2-binding sites in the 3′-UTR, and a plasmid expressing either MS2 protein or MS2-fusion, as indicated. Firefly/Renilla ratios were calculated. Relative luciferase activity represents the ratio of the reporter containing MS2-binding sites to the reporter lacking a site. Normalized signals for the MS2 control were set to 1 ( b ) Tethering assays in wild-type V6.5 ESCs were performed as in ( a ) except Rck, TNRC6B, or Trim71 not fused to MS2 (and hence not tethered to the firefly luciferase mRNA 3′-UTR). ( c ) Tethering assays in Hela cells performed as in ( a ) with the indicated Trim71 deletion MS2 fusion proteins. Normalized signals for the MS2 control were set to 1. Error bars represent mean +/−s.d. with n =3. The P -values are from two-tailed t -test result. NS = not significant. ( d ) Schematic representation of functional domains of Trim71. Full size image Trim71 is critical for rapid ESC proliferation Our results indicate that Trim71 functions with the miR-290 and miR-302 families to repress Cdkn1a expression in ESCs. Therefore, we next tested the role of Trim71 in ESC proliferation. Trim71 knockdown led to decreased cell numbers compared with a control siRNA ( Fig. 8a ). To exclude the possibility that reduction of Trim71 may increase cell death, we examined the number of cells undergoing apoptosis by propidium iodide and fluorescein isothiocyanate (FITC)-conjugated Annexin V staining. We found no significant difference between the control and Trim71-depleted cells (data not shown). Conversely, Trim71 overexpression resulted in increased cell numbers compared with a control plasmid ( Fig. 8b ). In the aforementioned Trim71 overexpression studies, we are able to detect mCherry::Trim71 expression in ~30% of the transfected ESCs (not shown). Collectively, these data strongly support a role for Trim71 in promoting rapid proliferation of ESCs. 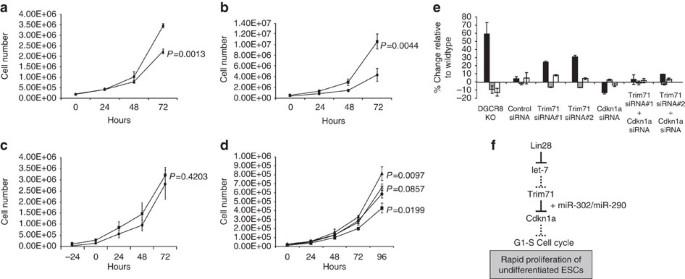Figure 8: Trim71 facilitates the cell cycle G1–S transition to promote rapid ESC proliferation. (a–d) ESCs were transfected with the indicated expression vectors or siRNAs Trim71 (siRNA#2). Equal numbers of cells were plated and cells counted daily starting from 48 h post-transfection (except for (c) that is starting from 24 h). Error bars represent mean +/−s.d. of biological triplicates. TheP-values are from two-tailedt-test result. (a) Trim71 depletion in J1 ESCs. Circles = control knockdown; Triangles = Trim71 knockdown. (b) Trim71 overexpression in V6.5 ESCs. Circles = control vector; Squares = Trim71 overexpression. (c) Trim71 overexpression in Dgcr8 KO ESCs. Circles = control vector; Squares = Trim71 overexpression. (d) Knockdown in J1 ESCs. Circles = control siRNA; Squares = Trim71 siRNA; Triangles = Cdkn1a siRNA; Crosses = Trim71 siRNA + Cdkn1a siRNA. (e) Cell cycle profile analysis of DGCR8 knockout ESCs, V6.5 ESCs (WT), and V6.5 transfected with siRNA targeting Trim71, Cdkn1a, or both. For each phase of the cell cycle, the data is presented as the percent change in populations compared with untransfected V6.5 ESCs. G1-phase (black bars); S-phase (gray bars); G2/M-phase (white bars). (f) Model of a Trim71 pathway in ESCs that leads to unrestricted cell cycle G1–S transition. Dashed lines indicate steps that are blocked in ESCs. Figure 8: Trim71 facilitates the cell cycle G1–S transition to promote rapid ESC proliferation. ( a – d ) ESCs were transfected with the indicated expression vectors or siRNAs Trim71 (siRNA#2). Equal numbers of cells were plated and cells counted daily starting from 48 h post-transfection (except for ( c ) that is starting from 24 h). Error bars represent mean +/−s.d. of biological triplicates. The P -values are from two-tailed t -test result. ( a ) Trim71 depletion in J1 ESCs. Circles = control knockdown; Triangles = Trim71 knockdown. ( b ) Trim71 overexpression in V6.5 ESCs. Circles = control vector; Squares = Trim71 overexpression. ( c ) Trim71 overexpression in Dgcr8 KO ESCs. Circles = control vector; Squares = Trim71 overexpression. ( d ) Knockdown in J1 ESCs. Circles = control siRNA; Squares = Trim71 siRNA; Triangles = Cdkn1a siRNA; Crosses = Trim71 siRNA + Cdkn1a siRNA. ( e ) Cell cycle profile analysis of DGCR8 knockout ESCs, V6.5 ESCs (WT), and V6.5 transfected with siRNA targeting Trim71, Cdkn1a, or both. For each phase of the cell cycle, the data is presented as the percent change in populations compared with untransfected V6.5 ESCs. G1-phase (black bars); S-phase (gray bars); G2/M-phase (white bars). ( f ) Model of a Trim71 pathway in ESCs that leads to unrestricted cell cycle G1–S transition. Dashed lines indicate steps that are blocked in ESCs. Full size image DGCR8-deficient ESCs lack mature miRNAs, display a slow growth rate and have an extended population-doubling time [33] . We overexpressed Trim71 in DGCR8-deficient ESCs. Importantly, unlike in wild-type ESCs, we observed no significant difference in cell numbers between the control and Trim71-overexpressing cell populations, even though we typically detect comparable levels of ectopic Trim71 expression in both wild-type and miRNA-deficient transfected ESCs ( Fig. 8c , data not shown). This finding indicates that Trim71 requires miRNA activity to promote ESC proliferation. Finally, we tested whether Trim71 enhances cell proliferation by maintaining low levels of Cdkn1a in ESCs. Depletion of Trim71 slowed cell proliferation, and cells depleted of Cdkn1a displayed an accelerated growth rate. Importantly, the slowed proliferation phenotype caused by depletion of Trim71 was rescued by simultaneous depletion of Cdkn1a ( Fig. 8d ). We conclude that Trim71-mediated repression of Cdkn1a is a key regulatory event for rapid ESC cell cycle and proliferation. Trim71 promotes G1 to S transition in ESCs We next investigated the cell cycle profile of ESCs that have been depleted of Trim71, Cdkn1a, or both ( Fig. 8e ). As a control, we used DGCR8-deficient ESCs that accumulate in the G1 phase of the cell cycle [7] . When compared with wild-type ESCs, DGCR8-deficient ESCs showed a ~60% increase in the proportion of cells in G1 phase and a ~10% decrease in the proportion of cells in both S and G2/M phases. Interestingly, Trim71-depleted ESCs also showed a significant increase (25–31%) in the proportion of cells in G1 phase compared with control knockdown cell populations, and a concomitant decrease (6–7%) in S phase. On the other hand, cell populations depleted of Cdkn1a exhibited the opposite effect, an ~13% decrease in G1 phase and a ~3% increase in S phase. Finally, simultaneous knockdown of Trim71 and Cdkn1a restored the cell cycle profile to that of wild-type populations. In conclusion, this analysis reveals that Trim71 is critical for cell cycle control in ESCs, and Trim71 facilitates the transition from G1 to S phase by repressing Cdkn1a expression. We investigated the molecular and cellular function of Trim71 in mouse ESCs. We found that Trim71 associates with Ago2 together with ESC-specific miRNAs and localizes to P-bodies. We found that the NHL domain of Trim71 and miRNAs are required for the interaction with Ago2, and multiple domains, including the NHL repeats, mediate Trim71 subcellular localization to P-bodies. We also found that the Trim71-containing ribonucleoprotein complex cooperates with ESC miRNAs to post-transcriptionally repress expression of the cell cycle regulator Cdkn1a. We furthermore identify the coiled-coil as a domain required for PTGS when tethered to a reporter mRNA. We conclude that Trim71-mediated repression of Cdkn1a is central to the characteristic expedited G1–S transition and rapid proliferation of ESCs. The expedited G1–S transition in the ESC cell cycle endows them with a highly proliferative capability, which reflects rapid growth during early embryogenesis. Progression through the G1–S phase in ESCs is primarily controlled by the constitutive activity of the cyclin E-Cdk2 complex. Cdkn1a, a member from the Cip/Kip family of cyclin-dependent kinase (Cdk) inhibitor proteins, is the key inhibitor of the cyclin E-Cdk2 complex [34] . We identify that Trim71 is required to maintain low levels of Cdkn1a expression in ESCs. We propose a model in which miRNAs and Ago2 function to recruit Trim71 to target mRNAs including Cdkn1a. Our demonstration that the NHL domain of Trim71 is required for this interaction is consistent with other Trim-family members including Drosophila Brat, Mei-P26 and Dappled that have been reported to interact with Ago1 (ref. 25 . Moreover, Trim32 potentiates miRNA function via its NHL domain, and the NHL domain of Brat mediates the recruitment of Brat to hunchback (hb) mRNA (via protein–protein interactions with other RNA-binding proteins) to induce hb translational repression [35] , [36] . Interestingly, the majority of loss-of-function mutations for the C. elegans lin-41 gene reside in its NHL domain [19] . We further show that the Trim71 interaction with Ago2 is mediated by mature miRNAs. Indeed, a miRNA-binding deficient Ago2 mutant (Ago2-PAZ10) fails to associate with Trim71. We emphasize that the increased proliferation in ESCs overexpressing Trim71 requires miRNAs, as ectopic Trim71 expression in DGCR8-deficient ESCs does not lead to changes in cell proliferation. We also note that Trim71-depleted ESCs exhibit a similar proliferation defect to the miRNA-deficient ESCs [33] . Altogether, our data strongly indicate that Trim71 functions with the ESC-specific miRNAs to sustain a rapid cell cycle in ESC, which is further supported by the genetic interaction of Trim71 and Cdkn1a in cell proliferation ( Fig. 8d ) and cell cycle analyses ( Fig. 8e ). We note that, unlike all other NHL-containing proteins that have been characterized, which reportedly inhibit stem cell proliferation and promote differentiation, our data establishes a role for Trim71 as a positive regulator of stem cell proliferation. Lin28 functions to inhibit the maturation of let-7 miRNAs in undifferentiated cells and may be important for both establishment and maintenance of ESC self-renewal and pluripotency [10] . We have confirmed that Trim71 is a bona fide let-7 target. As Lin28 inhibits let-7 expression, Trim71 levels are dependent on Lin28 expression, and accordingly, we find that depletion of Lin28 leads to substantial decrease in Trim71 protein levels. In light of our data, we propose that in ESCs Lin28 functions to maintain a low let-7 level that permits expression of Trim71. Trim71 cooperates with ESC-specific miRNAs to inhibit expression of Cdkn1a and promote rapid ESC proliferation ( Fig. 8f ). A report by Rybak et al . suggests that Trim71 functions as an E3 ubiquitin ligase that induces degradation of Ago2 and interferes with silencing of targets for let-7 and miR-124 miRNAs [22] . They propose a model in which Trim71 cooperates with Lin28 in suppressing let-7 activity. In contrast, however, we do not detect changes in Ago2 levels on Trim71 knockdown. Our findings indicate a different mechanism whereby Trim71 functions downstream of Lin28 to sustain ESC self-renewal. As overexpression of Lin28 (ref. 37 ), introduction of ESC-specific miRNAs, or knockdown of Cdkn1a can all lead to enhanced reprogramming of differentiated fibroblasts to induced pluripotent stem cells [38] , [39] , [40] , it will be interesting to explore the role of Trim71 in this context. Cell culture and cell lines HeLa and HEK293 were maintained in DMEM, P19 in MEMα+GlutaMax-1, and ESCs in DMEM with ESGRO (1,000 U ml −1 ), supplemented with antibiotics, and 10–15% fetal bovine serum. Dox-inducible Flag-Trim71 and Flag-Ago2 KH2 ESC lines were generated as per manufacturer's instructions (Open Biosystems) [41] . Embryoid bodies were formed by the hanging-drop method. Protein affinity purification KH2 ES cell lines were treated with Dox at 1 μg ml −1 for 72 h then collected in lysis buffer (20 mM Tris–HCl, pH 8.0, 137 mM NaCl, 1 mM EDTA, 1% (v/v) Triton X-100, 10% (v/v) Glycerol, 1.5 mM MgCl 2 , 1 mM DTT, 0.2 mM PMSF). Protein complexes were affinity-purified using α-Flag M2 agarose beads (Sigma) and washed 6X with EDTA-free BC-100 buffer (20 mM Tris, pH 7.6, 100 mM KCl, 10 mM β-Mercaptoethanol, 10% (v/v) Glycerol, 0.2% (v/v) Nonidet P-40, 0.2 mM PMSF) before elution with 0.5 mg ml −1 Flag peptide. For co-IP experiments with RNase A treatment, 20 μg ml −1 of RNase A was added to whole cell extracts or to the IP and incubated overnight at 4 °C (control samples were also treated as described but without RNase A). For IP, beads were washed 3X with EDTA-free BC buffer with the indicated KCl concentration, treated with 20 μg ml −1 of RNase A again (in EDTA-free BC-100 buffer) for 30 min at 37 °C, and washed 3 more times. DNA constructs Trim71 and Ago2 cDNAs were cloned into pBK-CMV vector (Stratagene) with an N-terminal Flag-tag and subcloned to pBS31 (Open Biosystems). Trim71 was additionally subcloned into the HindIII and XbaI sites of pFlag-CMV2 (Sigma) to generate pFlag-Trim71. For N-terminal deletions, PCR amplification was carried out using the forward primers ΔN147 5′-CATAAAGCTTAACCACCGGCACCATGCG-3′; ΔN302 5′-CATAAAGCTTGATGCCCTGCAGGACTCTC-3′; ΔN412 5′-CATAAAGCTTCGCGCCCTGGACATCCTG-3′; ΔN570 5′-CATAAAGCTTCGCAGCTACGTGGGCATCGG-3′ and the reverse primer 5′-GGGTCTAGATTAGAAGATGAGGATTCGATTG-3′. For C-terminal deletions, PCR amplification was carried out using the forward primer 5′-CATAAAGCTTATGGACTACAAAGACGATGACGAC-3′ and the reverse primers ΔC276 5′-GGGTCTAGAGGGGAGCCCGATGCCCACGTAGCT-3′; ΔC542 5′-GGGTCTAGAGATGGTGAGTGCCCGAGAGTCCTGC-3′. The N-terminal deletion ΔN69 was generated by subcloning the XhoI-SwaI fragment from pBK-Trim71 into the SalI-SmaI sites of pFlag-CMV2. The mCherry ORF was PCR amplified utilizing the forward (5′-CATAAAGCTTATGGTGAGCAAGGGCGAGGAGGATAAC-3′) and reverse (5′-CGATAAGCTTCTTGTACAGCTCGTCCATGCCGC-3′) primers and inserted into the HindIII site of pFlag-Trim71 full-length and deletion constructs. pGL3c (Promega) was digested with BglII and NcoI wherein the PCR product amplified from the TK promoter of pRL-TK (Promega) was inserted to generate pGL3c_TK. TK Promoter amplification was carried out using primers TKp Forward (5′-TAGCGAGATCTGGGGACCGTATACGTGGAC-3′) and TKp Reverse (5′-TAGCGCCATGGGGTGGCTAGCCTATAGTGAGT-3′). The luciferase reporter containing the segment of wild-type Cdkn1a 3′-UTR was generated by annealing the oligo pairs (forward primer: 5′-CTAGAGGGGGTGATCCTCAGACCTGAATAGCACTTTGGAAAAATGAGTAGGACTTTGGT-3′; reverse primer: 5′-CTAGACCAAAGTCCTACTCATTTTTCCAAAGTGCTATTCAGGTCTGAGGATCACCCCCT-3′) to obtain a 59-bp fragment, which was cloned into XbaI-linearized pGL3c_TK. The reporter containing mutant Cdkn1a 3′-UTR was generated by annealing the oligo pairs (forward primer: 5′-CTAGAGGGGGTGATCCTCAGACCTGAATGGATCAGTGGAAAAATGAGTAGGACTTTGGT-3′; reverse primer: 5′-CTAGACCAAAGTCCTACTCATTTTTCCACTGATCCATTCAGGTCTGAGGATCACCCCCT-3′). For the luciferase reporter containing the two let-7 binding sites from the Trim71 3′-UTR, the 204-bp PCR fragment (forward primer: 5′-AGCTACTCTAGAATTTCTTTTTCTTTTTCCCCCCCTTTAT-3′; reverse primer: 5′-AGCTACTCTAGACCTCCTAGGCCTTCAGGAG-3′) amplified from C57BL/6J genomic DNA was digested with XbaI, purified, and cloned into XbaI-linearized pGL3c_TK. For tethering assays, a luciferase reporter containing two copies of the MS2 binding site was generated by annealing the oligo pairs (forward primer: 5′-CTAGACGCGTACACGATCACGGTACGCTGAATTAGATCTCTGCGGATAGCATGAGGATCACCCATGCTCCCGGGGT-3′; reverse primer: 5′- CTAGACCCCGGGAGCATGGGTGATCCTCATGCTATCCGCAGAGATCTAATTCAGCGTACCGTGATCGTGTACGCG T-3′) to obtain a 72-bp fragment, which was then cloned into XbaI-linearized pGL3c_TK. The Rck ORF was amplified from cDNA using the forward 5′-CATAAAGCTTATGAGCACGGCCAGAACAGAGAAC-3′ and reverse 5′-GGGTCTAGATTACGGTTTCTCGTCTTCTGCAGGCTCACTGT-3′ primers and cloned into the HindII and XbaI sites of pFlag-CMV2. The C-terminal fragment of TNRC6B was cloned to generate pFlag-TNRC6B C-term [32] . MS2 ORF was PCR amplified from pEGFP-MS2-NLS, is from Dr Paul Anderson (forward primer: 5′-CATAAAGCTTATGGCTTCTAACTTTACTCAGTTCGTTC-3′; reverse primer: 5′-CGATAAGCTTGTAGATGCCGGAGTTTGCTGCGATTGC-3′) and cloned into the HindIII site of pFlag-CMV2, pFlag-Trim71, pFlag-Trim71 deletion constructs, pFlag-Rck, and pFlag-TNRC6B C-term to produce pFlag-MS2, pFlag-MS2–Trim71 (and deletion constructs), and pFlag-MS2-TNRC6B C-term, respectively. All constructs were confirmed by DNA sequencing. The Myc-Ago2-PAZ10 construct is from Dr Liu [4] . Luciferase assays were performed according to the Dual-luciferase Reporter Assay System protocol (Promega). Renilla luciferase-expressing vector (pRL-TK) was co-transfected for normalization. RNA Total RNA was isolated using TRIzol reagent (Invitrogen) except for mouse tissues (Ambion). For siRNA knockdown, the control siRNA (D-001810-01) and siGENOME siRNAs were purchased from Dharmacon. The target sequences are listed as follows: Trim71 siRNA #1 (D-161015-18), 5′-CAAGAAGAUGACCGCAUUA-3′; Trim71 siRNA #2 (D-161015-19), 5′-GGGCAAGAUCCUCGUUUCA-3′; Cdkn1a siRNA (D-058636-04), 5′-GGUGAUGUCCGACCUGUU C-3′; Lin28 siRNA, 5′-GGGUUG UGAUGACAGGCAA-3′. miRIDIAN miRNA hairpin inhibitors for negative control (IN-001005-01), mmu-let-7a (IH-310502-08), and mmu-miR-302a (IH-310483-07) were obtained from Dharmacon. Pre-miRNAs were purchased from Ambion. Cell transfections For transfection of DNA and RNA, Lipofectamine 2000 (Invitrogen) was used according to the manufacturer's instructions. Antibodies Antibodies. used for western blot: α-Trim71 (F4136, rabbit polyclonal) antibody was generated by Open Biosystems (immunogen sequence: KFGAQGSGFGQMDRPSGI) used at 1:1,000 dilution; β-Tubulin antibody (ab6046) used at 0.14 μg ml −1 , α-Sox2 (ab15830) used at 0.5 μg ml −1 , α-Nanog (ab21624) used at 0.2 μg ml −1 , and α-Oct4 (ab19857) used at 0.5 μg ml −1 from Abcam; α-Flag M2-Peroxidase (HRP) antibody (A8592) used at 0.4 μg ml −1 from Sigma; α-Ago2 antibody (C34C6, #2897) used at 1:1,000 dilution and α-Lin28A (A177, #3978) used at 1:1,000 dilution from Cell Signaling Technology; Mouse α-Cdkn1a (F-5, sc-6246) used at 1.0 μg ml −1 from Santa Cruz Biotechnology. mRNA and miRNA quantitative PCR For mRNA, 20 ng of total RNA was reverse transcribed using random hexamers and SuperScript III (Invitrogen). For miRNA, 5 ng of total RNA was reverse transcribed using gene-specific stem-loop RT primers and Multiscribe reverse transcriptase (Applied Biosystems). The resulting cDNAs were mixed either with iQ SYBR Green Supermix (Bio-Rad) (for mRNA), or with TaqMan Universal PCR Master Mix, No AmpErase UNG (Applied Biosystems) (for miRNA). Quantitative PCR was then performed using iCycler iQ Multicolor Real-Time PCR Detection System (Bio-Rad). Normalization controls include mouse β-actin for mRNAs and snoRNA142 for miRNAs. qRT–PCR Primers are listed: Trim71 forward: 5′-AATCACCGCGTGCAGATGTTTGAG-3′, reverse: 5′-AAGTCCACCACGACGATCAATCCA-3′; Oct-4 forward: 5′-ATCAGCTTGGGCTAGAGAAGGATG-3′, reverse: 5′-AAAGGTGTCCCTGTAGCCTCATAC-3′; Cdkn1a forward: 5′-CGAGAACGGTGGAACTTTGAC-3′, reverse: 5′-CAGGGCTCAGGTAGACCT TG-3′;. β-actin forward: 5′-CAGAAGGAGATTACTGCTCTGGCT-3′, reverse: 5′-TACTCCTGCTTGCTGATCCACATC-3′. In vitro slicer assays Reactions with Flag-purified proteins contained 0.5 nM. 5′-end labelled target RNA for miR-295 (5′-AGACUCAAAAGUAGUAGCACUUU-3′) or miR-302a (5′-UCACCAAAACAUGGAAGCACUUA-3′), 3.2 mM MgCl 2 , and 0.2 unit ml −1 RNaseOUT (Invitrogen). EDTA-free BC-100 was included in the reaction to bring the final volume to 30 μl. Samples were incubated at 37 °C for 60–90 min before analysis on a 15% (w/v) TBE-Urea gel. Immunohistochemistry KH2 cells were transfected with a DCP1a::GFP construct [4] cultured for 72 h on glass coverslips, and fixed for 20 min with 4% formaldehyde. After fixation, cells were washed with PBS followed by permeabilization and blocking using PBS containing 0.2% Triton X-100 and 5% donkey serum. Coverslips were incubated overnight at 4 °C in blocking solution containing α-Trim71 primary antibody (1:800). Cells were subsequently washed with 0.2% Triton X-100 in PBS, and incubated with a solution containing 1:1,000 donkey α-rabbit IgG secondary antibody (coupled to Alexa fluor 594, Invitrogen) and 1:2,000 4′,6-diamidino-2-phenylindole, dihydrochloride (DAPI, Invitrogen) for 1 h at room temperature. Cells were then washed with 0.2% Triton X-100 in PBS and mounted. HeLa cells were co-transfected with DCP1a::GFP and mCherry::Trim71 constructs, cultured for 48 h on glass coverslips and fixed for 20 min with 4% formaldehyde, washed with PBS and mounted. Cell proliferation and cell cycle analyses For cell proliferation assays, cells were counted daily beginning at 48 h post-transfection using Automatic Cellometer Reader (Nexcelom Bioscience). Cell apoptosis assays were performed using the Annexin V-FITC Apoptosis Detection Kit (BioVision). For cell cycle analysis, V6.5 (WT), DGCR8-null, and transfected V6.5 cells were cultured to ~60% confluence. Cells were trypsinized and single cell suspensions were prepared in cold PBS (1.5×10 6 cells ml −1 ). 1 ml of cells from each sample was then fixed by adding 3 ml of −20 °C absolute ethanol dropwise. After overnight fixation at 4 °C, the cells were washed with cold PBS twice, pelleted, and resuspended in 1-ml staining solution (1 mg ml −1 sodium citrate, 0.3% Triton X-100, 100 μg ml −1 propidium iodide, and 20 μg ml −1 ribonuclease A). Samples were stained for 30 minutes at room temperature before being analysed by flow cytometry. The cell cycle data were analysed by FlowJo using the Watson Pragmatic model (Cytometry 8:1–8) to define G1, S and G2/M phases. How to cite this article: Chang, H.-M. et al . Trim71 cooperates with microRNAs to repress Cdkn1a expression and promote embryonic stem cell proliferation. Nat. Commun. 3:923 doi: 10.1038/ncomms1909 (2012).